Optical virtual imaging at 50 nm lateral resolution with a white-light nanoscope The imaging resolution of a conventional optical microscope is limited by diffraction to ∼ 200 nm in the visible spectrum. Efforts to overcome such limits have stimulated the development of optical nanoscopes using metamaterial superlenses, nanoscale solid immersion lenses and molecular fluorescence microscopy. These techniques either require an illuminating laser beam to resolve to 70 nm in the visible spectrum or have limited imaging resolution above 100 nm for a white-light source. Here we report a new 50-nm-resolution nanoscope that uses optically transparent microspheres (for example, SiO 2 , with 2 μm<diameter<9 μm) as far-field superlenses (FSL) to overcome the white-light diffraction limit. The microsphere nanoscope operates in both transmission and reflection modes, and generates magnified virtual images with a magnification up to ×8. It may provide new opportunities to image viruses and biomolecules in real time. Optical microscopy is one of the most important scientific achievements in the history of mankind. It has revolutionized the field of life sciences and remains indispensible in many areas of scientific research. However, because of the diffraction limit, the imaging resolution of a classical optical microscope is limited to about half of the illuminating wavelengths λ . The root of the diffraction limit stems from the loss of evanescent waves in the far-field. These evanescent waves carry high spatial frequency subwavelength information of an object and decay exponentially with distance. In 2000, Pendry [1] proposed a theoretical 'superlens' that produces perfect diffraction-free images. Such superlenses are engineered from a slab of artificial negative-refraction medium in which the evanescent waves, instead of decaying, are enhanced across the slab. This offers the possibility to restore the nanoscale information in the far-field and therefore a nearly perfect image can be recovered [1] . The first laboratory optical superlens was made of a thin slab of silver material. Through the resonant coupling of evanescence waves to surface plasmon polaritons (SPP) in silver, objects as small as 60 nm were successfully recorded on a near-field photoresist layer in the ultraviolet spectrum ( λ /6 near-field resolution at λ =365 nm) [2] . Soon after, a SiC superlens working at mid-infrared frequency range ( λ =11 μm, λ /20 near-field resolution) was demonstrated to resolve 540 nm holes [3] . However, these superlenses are 'near-sighted', as the images can only be picked up in the near-field [4] . To project a near-field image into the far-field, a far-FSL was shortly proposed and demonstrated [5] , [6] . The FSL used a silver slab to enhance the evanescent waves and an attached line grating to convert the evanescent waves into propagating waves in the far-field. The FSL did not magnify objects. An approach to the making of a magnifying superlens is to use two-dimensional SPP confined by a concentric polymer grating placed on a gold surface. It generates a ×3 magnification and a resolution of 70 nm at 495 nm wavelength ( λ /7 far-field resolution) [7] . Hyperlens is another type of magnifying superlens. The hyperlens uses an anisotropic medium with a hyperbolic dispersion that generates a magnification effect through cylindrical or spherically curved multilayer stacks [5] , [8] , [9] . The hyperlens resolution reached 130 nm for 365 nm ultraviolet wavelength ( λ /3 far-field resolution) and 160 nm for 410 nm visible wavelength ( λ /2.6 far-field resolution), both with less than ×3 magnification [9] . Because of the SPP energy loss and sophisticated nanofabrication process, the resolutions of existing SPP superlens and hyperlens are limited at about ( λ /3– λ /7) within the visible spectrum. The other practical limit is that the SPP superlenses must be excited/illuminated with a specific laser source and parameter configurations (wavelength, polarization and incident angle). These superlenses would not function under a standard white-light source. Furthermore, the specific laser source required for SPP excitation could heat up, absorbing samples and damaging them. Heating due to SPP loss in superlenses could be another undesired effect that affects target materials in optical imaging [10] . It is therefore of significant appeal for scientists and engineers to develop a white-light optical nanoscope that works across the visible spectrum. In contrast to the SPP superlens, nanolenses (thickness<800 nm, diameter<3 μm) in plano-spherical-convex shape made of dielectric materials, for example, calix hydroquinone, are naturally loss-free and have been recently fabricated using sophisticated techniques for subwavelength imaging. These nanolenses were nanoscale solid immersion lenses (nSILs) [11] that resolve 220 nm line objects at 475 nm imaging wavelength ( λ /2.2 far-field resolution, ×2 magnification) [12] . Compared with macroscopic SILs, wavelength-scale nSILs can produce a 25% smaller focus spot, which enhances the resolution [11] . However, it remains practically impossible for SILs to resolve nano-objects below 100 nm with visible light sources on the basis of solid immersion mechanism due to the shortage of high-index lens materials [11] , [12] . In this study, we present a new 50-nm-resolution optical nanoscope that uses ordinary glass microspheres ( n =1.46, 2 μm<diameter<9 μm) as FSL to overcome the white-light diffraction limit, attaining a resolution between λ /8 and λ /14 (far-field resolution) and a magnification between ×4 and ×8. Such a super-resolution white-light nanoscope would open up new opportunities for imaging viruses, DNA and molecules in real time. 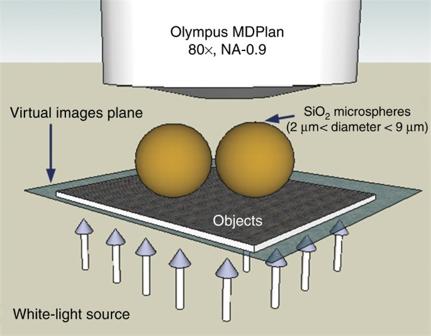Figure 1: Experimental configuration of white-light microsphere nanoscope withλ/8–λ/14 imaging resolution. Schematic of the transmission mode microsphere superlens integrated with a classical optical microscope. The spheres collect the near-field object information and form virtual images that can be captured by the conventional lens. Microsphere nanoscope and experimental imaging performance Figure 1 illustrates the schematic of a transmission mode white-light microsphere nanoscope. The microspheres are placed on the top of the object surface by self-assembly [13] . A halogen lamp with a peak wavelength of 600 nm is used as the white-light illumination source. The microsphere superlenses collect the underlying near-field object information, magnify it (forming virtual images which keep the same orientation as the objects in the far-field) and pick it up by a conventional ×80 objective lens (numerical aperture NA=0.9, Olympus MDPlan). In the experiments, gratings consisting of 360-nm-wide lines, spaced 130 nm apart, were imaged using 4.74-μm-diameter microspheres ( Fig. 2a ). The virtual image plane was 2.5 μm beneath the substrate surface and inside substrate. 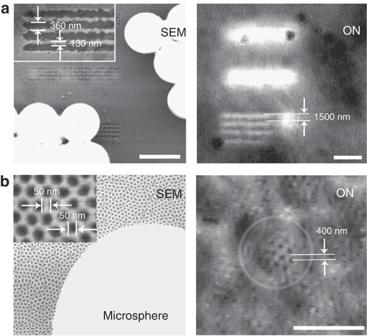Figure 2: Microsphere superlens imaging in transmission mode. (a) Microsphere superlens imaging of 360-nm-wide lines spaced 130 nm apart (top left image taken by scanning electron microscope (SEM)), the optical nanoscope (ON) image (top right image) shows that the lines are clearly resolved. (b) A gold-coated fishnet AAO sample imaged with a microsphere (a=2.37 μm, borders of two spheres are shown by white lines) superlens. The nanoscope clearly resolves the pores that are 50 nm in diameter and spaced 50 nm apart (bottom left SEM image). The size of the optical image between the pores within the image plane is 400 nm (bottom right ON image). It corresponds to a magnification factor ofM≈8. Scale bar, 5 μm. As can be seen from Figure 2a , only those lines with particles on top of them have been resolved. The lines without particles on top mix together and form a bright spot, which cannot be directly resolved by the optical microscope because of the diffraction limit (for the lowest visible wavelength λ =400 nm, the best diffraction-limited resolution is estimated to be 215 nm in air using the vector theory of Richards and Wolf [14] , and to be 152 nm by taking the solid immersion effect of a particle into account. For the main peak of a white-light source at λ =600 nm, the limits are 333 nm in air and 228 nm with solid immersion effect, respectively. Here, one should also note that the focal planes for lines with and without particles on top are different). The magnified image in Figure 2a corresponds to a ×4.17 magnification factor. Figure 2b shows a fishnet gold-coated anodic aluminium oxide (AAO) membrane imaged with 4.74-μm-diameter microspheres. The pores are 50 nm in diameter and spaced 50 nm apart. As it can be seen, the microsphere nanoscope resolves these tiny pores that are well beyond the diffraction limit, giving a resolution of between λ /8 ( λ =400 nm) and λ /14 ( λ =750 nm) in the visible spectrum range. It is important to note that the magnification in this case is around ×8, which is almost two times of that in the grating samples as shown in Figure 2a . This implies that the performance of microsphere superlens is affected by the near-field interaction of the sphere and the substrate. In our experiment, we have confirmed that the gold coating layer on the AAO surface not only enhanced the resolving power but also increased the magnification factor of the microsphere superlens. As self-assembled particles are easy to spread over a large surface area and meanwhile each particle can work as a superlens, the images produced by each particle can be stitched together to form a large image. These are the cases seen in Figure 2a,b , in which a hexagonal array of particles functions as an array of superlens covering a large area. Figure 1: Experimental configuration of white-light microsphere nanoscope with λ /8– λ /14 imaging resolution. Schematic of the transmission mode microsphere superlens integrated with a classical optical microscope. The spheres collect the near-field object information and form virtual images that can be captured by the conventional lens. Full size image Figure 2: Microsphere superlens imaging in transmission mode. ( a ) Microsphere superlens imaging of 360-nm-wide lines spaced 130 nm apart (top left image taken by scanning electron microscope (SEM)), the optical nanoscope (ON) image (top right image) shows that the lines are clearly resolved. ( b ) A gold-coated fishnet AAO sample imaged with a microsphere ( a =2.37 μm, borders of two spheres are shown by white lines) superlens. The nanoscope clearly resolves the pores that are 50 nm in diameter and spaced 50 nm apart (bottom left SEM image). The size of the optical image between the pores within the image plane is 400 nm (bottom right ON image). It corresponds to a magnification factor of M ≈8. Scale bar, 5 μm. Full size image Our previous calculations reveal the fact that the Poynting vector of the radiation reflected by the surface transfers through the particle [15] , which permits the formation of an image in the reflection mode as well. 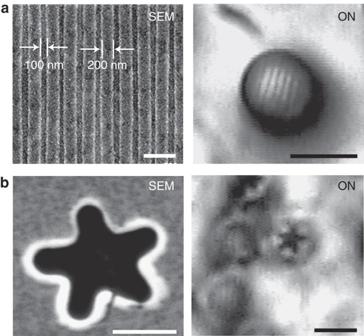Figure 3: Microsphere nanoscope reflection mode imaging. (a) Microsphere superlens reflection mode imaging of a commercial Blu-ray DVD disk. The 100-μm-thick transparent protection layer of the disk was peeled off before using the microsphere (a=2.37 μm). The subdiffraction-limited 100 nm lines (top left SEM image) are resolved by the microsphere superlens (top right ON image). (b) Reflection mode imaging of a star structure made on GeSbTe thin film for DVD disk (bottom left SEM image). The complex shape of the star including 90 nm corner was clearly imaged (bottom right ON image). Scale bar: SEM (500 nm), ON (5 μm). Figure 3a demonstrates a Blu-ray DVD disk (200-nm-wide lines separated 100 nm apart) imaged with 4.74-μm-diameter microspheres in the reflection mode using the halogen light illumination. The subdiffraction-limited lines are clearly observed. Figure 3b shows another example of reflection mode imaging of a star structure made on SbTe DVD disk. The complex shape of the star, including the 90 nm corners of the star, was clearly resolved by the microsphere superlens. Further experiments have confirmed that complex shape structures can also be well imaged in the transmission mode and that both the transmission and reflection modes can achieve 50 nm resolution. Indeed, the microsphere nanoscope has proven its practicability and versatility in nanoimaging of various samples. Figure 3: Microsphere nanoscope reflection mode imaging. ( a ) Microsphere superlens reflection mode imaging of a commercial Blu-ray DVD disk. The 100-μm-thick transparent protection layer of the disk was peeled off before using the microsphere ( a =2.37 μm). The subdiffraction-limited 100 nm lines (top left SEM image) are resolved by the microsphere superlens (top right ON image). ( b ) Reflection mode imaging of a star structure made on GeSbTe thin film for DVD disk (bottom left SEM image). The complex shape of the star including 90 nm corner was clearly imaged (bottom right ON image). Scale bar: SEM (500 nm), ON (5 μm). Full size image Experimental comparison with SILs imaging It is important to mention that we have also conducted comparison experiments using two SILs ( Supplementary Fig. S1 ), and confirmed that none of them can be used to resolve our samples with feature sizes between 50 and 130 nm ( Supplementary Fig. S2 ). Immersion of samples 'into' solids, attained by positioning the samples in close contact with the flat bottom surface of the lens, provides a means to access a shorter working wavelength in lens materials, and thus higher resolution beyond that in air. The resolution limit of the SILs used in our experiments was ∼ 152 nm, which makes it impossible to resolve the 100 nm objects. The imaging mechanism of the microsphere nanoscope In principle, the imaging resolution and magnification of the microsphere superlenses are fundamentally related to their focus properties [16] . It is well known that small spheres can generate 'photonic nanojets' with super-resolution foci [17] , less well known is that such super-resolution foci are only achievable for a narrow window of ( n , q ) parameters, where n is the refractive index of the sphere and q is the size parameter defined as q =2π a / λ , according to Mie theory [16] . 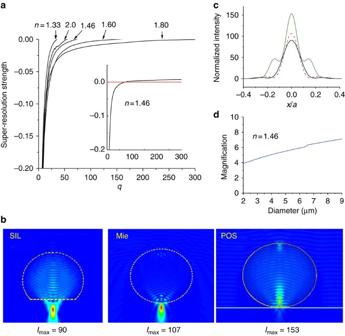Figure 4: Super-resolution foci and virtual magnification factor analyses. (a) Super-resolution strength, defined as (focus spot size−Rayleigh limit)/radius, as a function of size parameterqfor different refractive index particles. The inset showsqup to 300 forn=1.46. (b) The intensity distributions calculated for SIL (left image, heightH=a(1+n−1)), sphere (middle image) and particle on surface(right image) of a 40-nm-thick gold film for the sphere with radiusa=2.37 μm and refractive indexn=1.46 at the wavelengthλ=600 nm. (c) Full width at half maximum of foci for SIL (blue solid), sphere (red dot) and sphere on substrate (green solid). (d) Virtual image magnification versus particle size for sphere withn=1.46 at the wavelengthλ=600 nm. Figure 4a shows the calculated super-resolution window for different n and q parameters for spheres immersed in air. The y axis was calculated as (focus spot size−Rayleigh diffraction limit)/radius, which we name as super-resolution strength. For the n =1.46 spheres used in this study, super-resolution occurs for q <70, which corresponds to smaller than 9.0-μm-diameter spheres at a wavelength of λ =400 nm. From our experiments, it was verified that 10 and 50 μm spheres are not successful in 100-nm-resolution imaging tests, whereas 3.0 μm spheres produce clear 50-nm-resolution images as achieved by the 4.74 μm spheres. We also examined the use of 1 μm spheres for imaging. It is found that because of the small-view windows of such particles, high-resolution imaging was not successful. Therefore, the limit for 1 μm sphere is a practical conclusion rather than a theoretical one. The practical size window for n =1.46 microspheres is recommended as 2 μm<diameter<9 μm for 50-nm-resolution imaging. From Figure 4a , it can also be seen that refractive index has a strong effect on super-resolution foci; with n =1.8, the size window for super-resolution extends up to q ∼ 250, which implies that particles as big as 30 μm could be used for nanoimaging. This would facilitate the experiments because of wider view windows offered by bigger particles. Moreover, one can see that the super-resolution strength is maximized at n =1.8. When refractive index increases further to n =2.0, the super-resolution strength reduces and super-resolution window shrinks, making it undesirable to use n >1.8 high-index materials for nanoimaging in our technique. On the contrary, high-index ( n >1.8) materials are important for SILs as their imaging resolution is determined by the refractive index of lens materials because of the solid immersion mechanism. Figure 4: Super-resolution foci and virtual magnification factor analyses. ( a ) Super-resolution strength, defined as (focus spot size−Rayleigh limit)/radius, as a function of size parameter q for different refractive index particles. The inset shows q up to 300 for n =1.46. ( b ) The intensity distributions calculated for SIL (left image, height H = a (1+ n −1 )), sphere (middle image) and particle on surface(right image) of a 40-nm-thick gold film for the sphere with radius a =2.37 μm and refractive index n =1.46 at the wavelength λ =600 nm. ( c ) Full width at half maximum of foci for SIL (blue solid), sphere (red dot) and sphere on substrate (green solid). ( d ) Virtual image magnification versus particle size for sphere with n =1.46 at the wavelength λ =600 nm. Full size image Figure 4b,c compares the | E | 2 intensity distribution for SIL, sphere and particle on surface calculated with the same parameters, that is, n =1.46, diameter=4.74 μm and λ =600 nm. Here, one important difference between SIL and sphere was demonstrated: a super-resolution focus outside of sphere and a diffraction-limited focus for the same-diameter SIL. Truncating of sphere into SIL causes the loss of super-resolution focus, and diffraction-limited spot of SIL makes it impossible to resolve below 100 nm objects. Super-resolution foci are the key requirement of our technique. With the presence of a substrate, the focus at particle–substrate contact region generally becomes sharper. This is evidenced by our particle on surface calculation ( Fig. 4b,c ). Such effects could enhance the imaging resolution according to the reciprocity principle [18] . Magnification factor of the microsphere nanoscope In cases of macroscopic spheres and SILs, in which geometrical optics applies, the virtual image magnification factor can be calculated through ray tracing as M = f /( f − a ) for an object in contact with the lens surface, where f is the focal length and a is the distance between the object and the centre of the lens. Characteristically, spheres ( M ≈ n /(2− n )) produce a higher magnification over the SILs counterparts ( M ≈ n 2 ) for n <2.0 because of their shorter focal length f ( Supplementary Figs S3 and S4 ). As sphere size reduces to the super-resolution size window (2 μm<diameter<9 μm, n =1.46), geometrical ray tracing becomes invalid as evidenced by two signs. First, it fails to predict the magnification factor for those super-resolution spheres with f = a , as M = f /( f−a ) becomes infinite in these cases. Second, optical rays going through such small spheres could form optical vortices and singularities inside the sphere. ( Supplementary Figs S5 and S6 ). A mathematical model for near-field magnification with field singularities is still not available in literature. Here, we propose a fitting formula based on maximal field enhancement with some exponent, M ≈( I max / I 0 ) β . We found that the factor β ≈0.34 yields excellent agreement (<1% deviation) with exact virtual image magnification for geometrical optics approximation ( Supplementary Fig. S4 ). Using this simplified estimation, one can determine the magnification factor for the particle on surface to be M ≈5.5, which is in reasonable agreement with experimental values between 4 and 8 for different samples. In a similar manner, we found that magnification increases with particle size within super-resolution size window from M ≈4 for 2 μm spheres to M ≈7 for 9 μm spheres ( Fig. 4d ). The magnification-increasing tendency was also confirmed by experiments using 3.0 μm and 4.74 μm spheres; the magnification of 4.74 μm is about 1.2 times that of 3.0 μm spheres. The microsphere nanoscope demonstrated by us has a far-field resolution between λ /8 and λ /14 and a magnification between ×4 and ×8 Such resolution and magnification have greatly surpassed those of existing visible wavelength SPP hyperlens [7] , [8] (resolution λ /7, magnification ×2.4) and nSILs [11] , [12] (resolution λ /2.2, magnification ×2) within the visible spectrum; note that the SiC superlens resolution of λ /20, as demonstrated in the literature [3] , is not far-field resolution but a near-field resolution in mid-infrared spectrum range. The microsphere superlenses operate in a virtual imaging mode, and can be easily integrated with an ordinary optical microscope in both transmission and reflection modes, and work under a standard white-light illumination. From our estimations, it follows that maximal virtual image magnification can be attained with a refractive index n ≈1.8. With 5 μm particles, it should resolve arbitrary structures <20 nm, making it possible to directly observe viruses and the inside of living cells under white light without the need to excite fluorescence using proper lasers as in molecular fluorescence nanoscopy [19] . As a final note, particles in other shapes, such as elliptical particles, could also be considered for below 50 nm imaging as near-field foci strongly depend on particle shape. In conclusion, we have demonstrated that optically transparent microspheres are high-performance optical superlens that could resolve 50 nm objects by near-field virtual imaging under a white-light source illumination. The microsphere nanoscope is robust, economical and is also easy to accommodate different kinds of samples with potential applications for imaging biological objects such as virus, DNA and molecules. Imaging samples fabrication and preparation The gratings used in Figure 2a were fabricated using a focused ion beam machine (Quanta 200 3D, FEI). The sample consists of 30-nm-thick chrome film coated on fused silica substrates. The AAO used in Figure 2b was fabricated by two steps anodizing in oxalic acid (0.3 mol l −1 ), under a constant voltage of 40 V. A porous 20-nm-thick metallic film (gold) was then formed by using a 300-μm-thick AAO as the template. The star sample used in Figure 3b was fabricated using contact particle lens array technique, which was developed by us recently [20] . The diluted SiO 2 sphere suspension was applied onto the substrate surface by drop coating. The colloidal silica spheres (Bangs Laboratories) form an ordered monolayer through self-assembly. An Olympus microscope (MX-850), fitted with an ×80 objective lens (numerical aperture NA=0.9, Olympus MDPlan) was used to focus through the microsphere into the substrate and virtual images were collected and reported. All scanning electron microscopic images were taken by Hitachi S-3400N. SILs imaging Both 2.5-mm-diameter and 0.5-mm-diameter fused silica half-ball SILs) from Edmund Optics have been used for the control experiments ( Supplementary Fig. S1 ). The SILs were placed directly onto imaging sample surface by careful manual handling, attaining an experimental configuration similar to that for the microsphere. An ×80 objective lens was used for the 0.5-mm-diameter SIL and a ×40 lens for the 2.5-mm-diameter SIL, as limited by the available gap between lens and sample. All samples as in Figures 2 and 3 have been tested with SILs without success. Example results on Blu-ray disk imaging without SILs and particles, with 0.5 mm SIL, with 2.5 mm SIL and with 4.74 μm sphere were shown for comparison in Supplementary Figure S2 . Simulation method The geometrical optical ray tracing analysis ( Supplementary Fig. S3 ) was carried out using Mathematica 7.0 software, and field distributions in Figure 4 were calculated by Mie theory for sphere and finite difference in time domain technique for SIL and sphere and particle on surface, respectively. Virtual image magnification factor Magnification factor for virtual image can be found by ray tracing under the approximation of geometrical optics ( Supplementary Fig. S3 ). The focal lengths of SIL and sphere are f SIL ≈ an 2 /( n 2 −1) and f sphere ≈ na /2( n −1), respectively, where a is the radius. If a small point object A is situated at the plane of SIL at y A = y 0 ≪ a , then y image ≈ n 2 y 0 , that is, magnification of the virtual image is M SIL ≈ n 2 . At similar conditions, magnification of the virtual image by the sphere is presented by M sphere ≈ n /(2− n ). Thus, the spherical particle everywhere produces a higher magnification than SIL ( Supplementary Fig. S3 ). Following the focusing properties of the sphere under the approximation of geometrical optics [21] , the field enhancement in the focal area is given by Thus, under the approximation of geometrical optics, we have a relationship between field enhancement and magnification of virtual image, M sphere = f ( I max / I 0 ), written in a parametric form, where refractive index n has a role of parameter, see in Supplementary Figure S4 . This dependence with high accuracy can be approximated by a function M sphere ≈( I max / I 0 ) β , with β ≈0.34. The difference between the exact curve and approximated formula for M ( n ) is <1% for the whole range of refractive index from 1 to 1.95. Note that geometrical optics approximation yields singularity at n =2; thus, it cannot be applied in the vicinity of this point. Also, note that under the approximation of geometrical optics, field enhancement does not depend on the particle size. However, one can see this dependence under the approximation of the Mie theory, see Figure 4d in the article. Energy flow simulation Within the framework of classical Mie theory, the time-averaged Poynting vector (energy flow) is given by and field lines are the solutions of the differential equation d x / S x =d y / S y . We developed a Fortran program based on Mie formulation, and in Supplementary Figure S5 , we present the Poynting vector lines for the microsphere with radius a =2.37 μm and refractive index n =1.46 illuminated by a plane wave with λ=600 nm. We can construct the virtual image, using the reciprocity principle and extrapolation of the Poynting vector, on the basis of this angle of vector line on the outer edge of the particle, see in Supplementary Figure S6 . This method, in fact, uses the same idea of virtual image construction as in geometrical optics. We extrapolate not the straight ray but plot tangential line to the lines with some curvature. This image construction yields a magnification of 2–4 times depending on the particular Poynting vector line. How to cite this article: Wang, Z. et al . Optical virtual imaging at 50 nm lateral resolution with a white-light nanoscope. Nat. Commun. 2:218 doi: 10.1038/ncomms1211 (2011).